Increased MAPK reactivation in early resistance to dabrafenib/trametinib combination therapy of BRAF-mutant metastatic melanoma One-third of BRAF-mutant metastatic melanoma patients treated with combined BRAF and MEK inhibition progress within 6 months. Treatment options for these patients remain limited. Here we analyse 20 BRAF V600 -mutant melanoma metastases derived from 10 patients treated with the combination of dabrafenib and trametinib for resistance mechanisms and genetic correlates of response. Resistance mechanisms are identified in 9/11 progressing tumours and MAPK reactivation occurred in 9/10 tumours, commonly via BRAF amplification and mutations activating NRAS and MEK2. Our data confirming that MEK2 C125S , but not the synonymous MEK1 C121S protein, confers resistance to combination therapy highlight the functional differences between these kinases and the preponderance of MEK2 mutations in combination therapy-resistant melanomas. Exome sequencing did not identify additional progression-specific resistance candidates. Nevertheless, most melanomas carried additional oncogenic mutations at baseline (for example, RAC1 and AKT3) that activate the MAPK and PI3K pathways and are thus predicted to diminish response to MAPK inhibitors. Therapy targeting the mitogen-activated protein kinase (MAPK) pathway with combined BRAF and MEK inhibition was recently approved by the Australian Therapeutic Goods Administration, and had accelerated approval by the USA Food and Drug Administration for the treatment of BRAF V600 -mutant metastatic melanoma. The randomized phase II study of the BRAF inhibitor dabrafenib combined with the MEK inhibitor trametinib significantly improved response rates (76 versus 54%), prolonged progression-free survival (PFS; 9.4 versus 5.8 months) and reduced skin toxicities compared with single-agent dabrafenib, in patients with BRAF V600 -mutant metastatic melanoma [1] . The phase III study of this combination versus dabrafenib (NCT01584648) demonstrated an improved PFS in the combination-treated cohort (hazard ratio 0.75, P =0.035) [2] and a phase III trial demonstrated an overall survival (OS) benefit for this combination compared with vemurafenib monotherapy (NCT01597908) [3] . Other BRAF and MEK inhibitor combinations, including vemurafenib combined with cobimetinib [4] (NCT01689519) and encorafenib (LGX818) combined with binimetinib (MEK162; ref. 5 ; NCT01909453), have been or are also being evaluated in ongoing clinical trials in BRAF V600 -mutant melanoma patients. Despite significant improvements in clinical outcomes and reports of long-term responses [6] , 50% of patients treated with dabrafenib combined with trametinib progress at 9–10 months, and resistance remains a barrier to better patient outcomes. Acquired resistance to BRAF inhibitor monotherapy is primarily driven by MAPK reactivation [7] , [8] , [9] , via BRAF copy number gains, aberrant BRAF splicing, mutations in NRAS or MEK1/2 and upregulation of receptor tyrosine kinases [10] , [11] , [12] , [13] . The role of MAPK signalling and the spectrum of alterations conferring resistance to combined BRAF and MEK inhibition remain unknown. Given that many BRAF inhibitor resistance mechanisms are sensitive to MEK inhibition, alone or in combination with BRAF inhibition [7] , [10] , [14] , [15] , MAPK-independent mechanisms of resistance might be anticipated to predominate in melanomas treated with combined BRAF/MEK inhibition. However, a study of five BRAF inhibitor-naive patients with acquired resistance to combined BRAF and MEK inhibition identified potential resistance mechanisms in three patients, including a MEK2 Q60P mutation, amplification of the BRAF gene and expression of a BRAF-splice variant lacking exons 2–10 (BRAF ex2–10Δ ) [16] . The MEK2 Q60P mutation and BRAF amplification have been shown to confer resistance to combined BRAF and MEK inhibition in preclinical models [16] . BRAF-splice variants, however, remain sensitive to MEK inhibition [7] , [12] , [14] , thus the contribution of BRAF ex2–10Δ in combination BRAF/MEK resistance remains unclear. Defining the mechanisms of acquired resistance to combined BRAF and MEK inhibition and how they may differ from those observed with single-agent BRAF inhibition may provide an opportunity for therapeutic exploitation, particularly in patients who show minimal clinical benefit. Here we describe resistance mechanisms in 20 melanoma samples (9 pre-treatment and 11 progressing (Prog) metastases) derived from 10 BRAF V600 -mutant melanoma patients who had early resistance to combined BRAF and MEK inhibitor therapy. 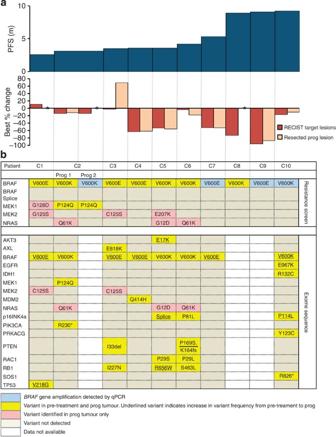Figure 1: Combination BRAF and MEK inhibition resistance mechanisms and clinical correlates. (a) PFS, best overall RECIST response and best Prog-specific RECIST response by mechanism of resistance to CombiDT (n=10). *Best response for Progs from patients C1, C2 and C8 was not obtained. (b) Spectrum of candidate resistance variants; Prog-specific (acquired) and variants found in both pre-treatment and Prog metastases. Patients and melanoma tissue samples Eleven Prog and nine matched pre-treatment melanoma tumour samples derived from 10 BRAF V600 -mutant melanoma patients treated with dabrafenib plus trametinib (CombiDT) were analysed ( Table 1 ). Two patients received prior MAPK pathway inhibitors; patient C10 received dabrafenib monotherapy and patient C3 received trametinib monotherapy. All patients were on CombiDT at the time of Prog biopsy, except patient C7 who had ceased treatment 1 month before resection. All characterized Prog tumours were pre-existing metastases that initially responded but subsequently progressed on combination therapy, except patients C1 and C3, whose Prog tumours had no clinical or radiographic response to CombiDT ( Fig. 1 ). The median RECIST response, RECIST response rate, median PFS and OS for this cohort were 35%, 50%, 3.9 months and 11.8 months, respectively ( Fig. 1 ), consistent with early resistance and poor clinical outcomes. Eight patients (C1 to C8) ceased CombiDT treatment after RECIST progression and none had evidence of tumour regression post-CombiDT cessation. Table 1 Patient, treatment outcome and resistance characteristics. Full size table Figure 1: Combination BRAF and MEK inhibition resistance mechanisms and clinical correlates. ( a ) PFS, best overall RECIST response and best Prog-specific RECIST response by mechanism of resistance to CombiDT ( n =10). *Best response for Progs from patients C1, C2 and C8 was not obtained. ( b ) Spectrum of candidate resistance variants; Prog-specific (acquired) and variants found in both pre-treatment and Prog metastases. Full size image Spectrum of acquired resistance mechanisms to combined BRAF and MEK inhibition An acquired resistance mechanism activating the MAPK pathway was identified in 9 of 11 Prog tumours (82%; Table 1 ; Fig. 1 ); BRAF amplifications were detected in 4 (36%), MEK1/2 mutations in 3 (27%) and oncogenic NRAS mutations in 3 (27%) Prog tumours ( Figs 1 and 2 ). None of these alterations were identified in the matched pre-treatment samples. 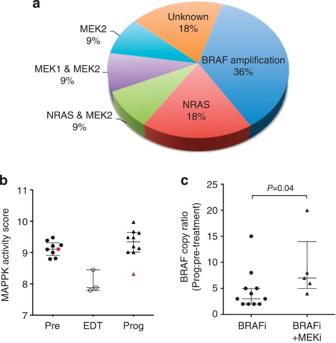Figure 2: MAPK signalling reactivated in combination-resistant Prog metastases. (a) Mechanisms of resistance in Prog tumours (n=11). (b) Box plots showing MAPK activity (mean log2-transformed expression of MAPK activation gene transcripts) in pre-treatment (Pre;n=9) and matched Prog tumours (n=10). The impact of MAPK inhibition on MAPK activity is also shown in three EDT tumours (EDT); one patient in this report (patient C1) and two previously reported BRAF inhibitor monotherapy patients7. Only the Prog sample derived from patient C5 (pre-treatment and matched Prog highlighted in red) showed significant downregulation of MAPK activity relative to the matched pre-treatment biopsy (NES=−1.91, false discovery rateq<0.001). MAPK activation gene set derived from ref.18. The median values and interquartile ranges are shown. (c) Box plot showing Prog to pre-treatment ratio ofBRAFgene copies in BRAF inhibitor (BRAFi)-resistant and combination-resistant (BRAFi+MEKi) Progs. Data were obtained from refs7,8,9,17. The median values and interquartile ranges are shown. Figure 2: MAPK signalling reactivated in combination-resistant Prog metastases. ( a ) Mechanisms of resistance in Prog tumours ( n =11). ( b ) Box plots showing MAPK activity (mean log2-transformed expression of MAPK activation gene transcripts) in pre-treatment (Pre; n =9) and matched Prog tumours ( n =10). The impact of MAPK inhibition on MAPK activity is also shown in three EDT tumours (EDT); one patient in this report (patient C1) and two previously reported BRAF inhibitor monotherapy patients [7] . Only the Prog sample derived from patient C5 (pre-treatment and matched Prog highlighted in red) showed significant downregulation of MAPK activity relative to the matched pre-treatment biopsy (NES=−1.91, false discovery rate q <0.001). MAPK activation gene set derived from ref. 18 . The median values and interquartile ranges are shown. ( c ) Box plot showing Prog to pre-treatment ratio of BRAF gene copies in BRAF inhibitor (BRAFi)-resistant and combination-resistant (BRAFi+MEKi) Progs. Data were obtained from refs 7 , 8 , 9 , 17 . The median values and interquartile ranges are shown. Full size image Ten Prog tumours underwent gene set enrichment analysis (GSEA) of gene expression; nine showed reactivation of MAPK activity signatures, that is, MAPK pathway signalling in these progressing lesions, biopsied while the patient was receiving CombiDT, was comparable to the matched pre-treatment melanoma tumours ( Table 1 ; Fig. 2b ). Significantly, the MAPK activity in these Prog tumours was substantially higher than MAPK activity in three early during treatment (EDT) tumours, consistent with early response to CombiDT followed by subsequent disease progression. Of the nine MAPK-reactivated Prog tumours, eight had an established mechanism of resistance and one (Prog derived from patient C4) had no identified resistance driver. The Prog that did not show evidence of MAPK reactivation by GSEA (patient C5; Fig. 2b ) had two identified resistance mechanisms (MEK2 E207K and NRAS G12D ; Supplementary Fig. 1 ), but both variants occurred at low frequency (13 and 15% allelic frequency, respectively, by whole-exome sequencing; Supplementary Fig. 2 ), suggesting heterogeneity within the Prog metastasis. Exome sequencing revealed an AKT3 E17K mutation present in both the pre-treatment and Prog metastases derived from patient C5 (see below) and immunohistochemistry analyses confirmed substantial pAKT expression in the Prog tissue and in the responding EDT metastasis resected at day 9 (pre-treatment tissue was not available for this analysis; Fig. 3 ). Similarly, heterogeneity was seen in the resected Prog from patient C1. One portion of the tumour screened by capillary sequencing of reverse transcription PCR (RT–PCR) products contained both the MEK1 G128D and MEK2 C125S mutations ( Supplementary Fig. 1 ) and demonstrated MAPK reactivation. In contrast, a second portion of the same tumour was exome sequenced and contained only the MEK2 C125S mutation (30% allele variant frequency; Supplementary Table 1 ). 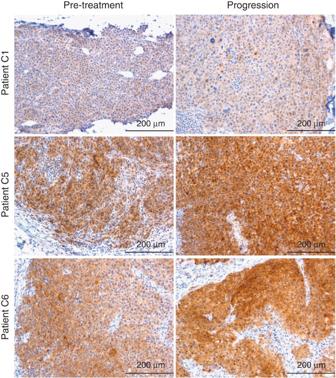Figure 3: Expression of pAKT in matched pre- or early-treatment and Prog tumours derived from patients C1, C5 and C6. High levels of phosphorylated AKT in the matched pre-treatment and Prog tumour samples derived from patients C5 and C6. AKT3E17Kand RAC1P29Smutations were identified in pre-treatment and Prog tumours derived from patient C5, and RAC1P129Land PTENK164fsmutations were identified in the pre-treatment and Prog tumours derived from patient C6. In contrast, AKT phosphorylation was low in the pre-treatment and Prog tumours derived from patient C1. These tumours had no detectable oncogenic PI3K-AKT pathway mutations. For patient C5, the EDT tumour (taken at day 9 of a CombiDT-responding lesion) is shown in place of a pre-treatment tumour. Figure 3: Expression of pAKT in matched pre- or early-treatment and Prog tumours derived from patients C1, C5 and C6. High levels of phosphorylated AKT in the matched pre-treatment and Prog tumour samples derived from patients C5 and C6. AKT3 E17K and RAC1 P29S mutations were identified in pre-treatment and Prog tumours derived from patient C5, and RAC1 P129L and PTEN K164fs mutations were identified in the pre-treatment and Prog tumours derived from patient C6. In contrast, AKT phosphorylation was low in the pre-treatment and Prog tumours derived from patient C1. These tumours had no detectable oncogenic PI3K-AKT pathway mutations. For patient C5, the EDT tumour (taken at day 9 of a CombiDT-responding lesion) is shown in place of a pre-treatment tumour. Full size image Selection of BRAF copy number gains and MEK2 alterations Gain of BRAF copy number was the most common mechanism for developing resistance to CombiDT, with 4/11 Prog tumours showing amplification encompassing the BRAF gene. This finding was unexpected given first the substantially lower incidence of BRAF amplification in tumours progressing on BRAF inhibitor monotherapy (18/140=13%) [7] , [8] , [9] , and second, preclinical studies showing that overexpression of BRAF in sensitive melanoma cells confers resistance to MEK inhibitor monotherapy, but they remain sensitive to combined BRAF and MEK inhibition [10] . We therefore examined the extent of BRAF amplification in several cohorts [7] , [8] , [9] , [17] , and, although the numbers of tumours available for analyses were small, we found a significant increase in the BRAF Prog to pre-treatment copy number ratio in CombiDT-resistant tumours compared with tumours progressing on BRAF inhibitor monotherapy ( P =0.04; Fig. 2c ). BRAF-splice variants have been identified as a mechanism of resistance to BRAF inhibitor monotherapy [7] , [8] , [12] . In contrast, no BRAF-splice isoforms were detected in the 11 CombiDT-resistant melanomas in this cohort. Analysis of patient-derived and in vitro -generated dabrafenib-resistant melanoma cell lines expressing endogenous BRAF-splice variants lacking exons 2–8, 2–10 and 4–10 (ref. 14 ) confirmed that these cells were resistant to dabrafenib monotherapy but retained sensitivity to single-agent trametinib ( Fig. 4a ). 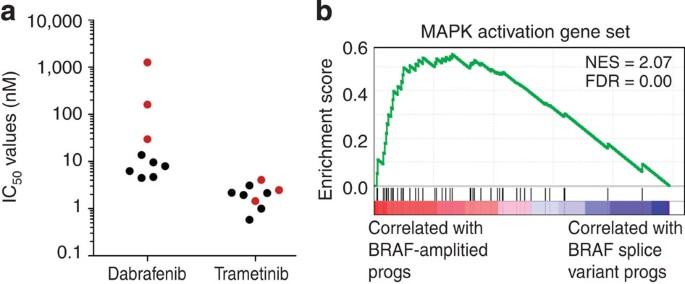Figure 4: BRAF-splice variants confer diminished BRAF inhibitor sensitivity, but remain sensitive to MEK inhibition. (a) IC50values of dabrafenib and trametinib in a panel of BRAF-mutant melanoma cell lines. The SMU027 and WMD009 patient-derived cells and BR4in vitrogenerated dabrafenib-resistant cell lines that express BRAF-splice isoforms (BRAFex2–8Δ, BRAFex2–10Δ, BRAFex4–10Δ; ref.14) and are highlighted in red. Other melanoma cells include NM176, MM200, M238, M249, SKMel28 and NM182 (black). (b) GSEA shows enrichment of MAPK activation gene set in Prog tumours withBRAFcopy number gains (n=5) versus Prog tumours with BRAF-splice isoforms (n=7). MAPK activation gene set derived from ref.18. The false discovery rate (FDR) statistic and normalized enrichment score (NES) are indicated. Figure 4: BRAF-splice variants confer diminished BRAF inhibitor sensitivity, but remain sensitive to MEK inhibition. ( a ) IC 50 values of dabrafenib and trametinib in a panel of BRAF-mutant melanoma cell lines. The SMU027 and WMD009 patient-derived cells and BR4 in vitro generated dabrafenib-resistant cell lines that express BRAF-splice isoforms (BRAF ex2–8Δ , BRAF ex2–10Δ , BRAF ex4–10Δ ; ref. 14 ) and are highlighted in red. Other melanoma cells include NM176, MM200, M238, M249, SKMel28 and NM182 (black). ( b ) GSEA shows enrichment of MAPK activation gene set in Prog tumours with BRAF copy number gains ( n =5) versus Prog tumours with BRAF-splice isoforms ( n =7). MAPK activation gene set derived from ref. 18 . The false discovery rate (FDR) statistic and normalized enrichment score (NES) are indicated. Full size image These apparent differences in BRAF gene alterations between tumours resistant to mono- or combination MAPK inhibition suggested that BRAF genetic alterations might differ in their activation of downstream MAPK signalling. We therefore examined MAPK signalling using an established gene transcription signature, indicative of persistent MAPK activation [18] . A comparison between five BRAF-amplified Progs (including one dabrafenib-resistant BRAF-amplified Prog tumour [7] ) and seven previously described BRAF-splice variant Prog tumours [7] confirmed significantly elevated MAPK signalling in the BRAF -amplified class (GSEA normalized enrichment score=2.07, false discovery rate q =0.00, P =0.00; Fig. 4b ). Mutations affecting MEK1 and MEK2 have each been identified in 8/154 (5%) and 5/154 (3%) of melanomas progressing on BRAF inhibitor monotherapy, respectively [7] , [8] , [9] . In comparison, we found that MEK2 alterations were predominant over MEK1 genetic alterations in CombiDT-resistant Progs (3/11=27%). The relative frequency of acquired MEK2 mutations was significantly increased in melanomas progressing on combination dabrafenib/trametinib (4/16; this report and ref. 16 ) compared with melanomas progressing on BRAF inhibitor monotherapy (5/154; Fisher’s exact test; P =0.01). Functional analyses of MEK1 and MEK2 mutant proteins with mutations in equivalent residues—MEK1 C121S versus MEK2 C125S —confirmed that, although both mutant MEK proteins displayed elevated ERK kinase activity, relative to the wild-type MEK protein ( Supplementary Fig. 3 ), only expression of the MEK2 C125S mutant (found in two combination-resistant Progs; patients C1 and C3) was associated with significant levels of phosphorylated retinoblastoma protein (a marker of cell proliferation), phosphorylated ERK and colony growth in the presence of combined dabrafenib and trametinib ( Fig. 5 ). 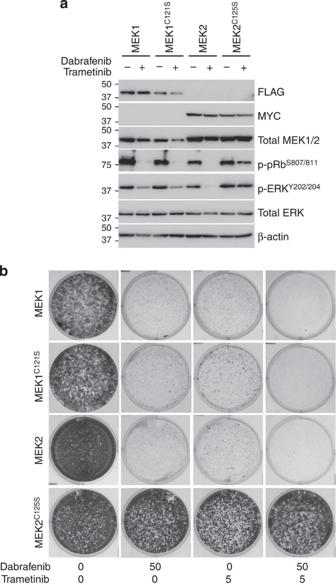Figure 5: MEK2C125S, but not the equivalent MEK1C121Svariant, confers robust resistance to dabrafenib and trametinib. (a) SKMel28 melanoma cells were stably transduced with the indicated MEK constructs. Cell lysates were analysed for the indicated proteins 48 h after incubation with dabrafenib (50 nM) and trametinib (5 nM). Ectopically expressed MEK1 and MEK2 proteins were tagged with the FLAG and MYC epitopes, respectively. (b) Transduced SKMel28 cells were seeded at low density and 24 h after seeding were treated with the indicated concentrations of dabrafenib and trametinib every 72–96 h. Colonies were stained with crystal violet 10 days post transduction. Photographs are representative of at least two independent transduction experiments. Figure 5: MEK2 C125S , but not the equivalent MEK1 C121S variant, confers robust resistance to dabrafenib and trametinib. ( a ) SKMel28 melanoma cells were stably transduced with the indicated MEK constructs. Cell lysates were analysed for the indicated proteins 48 h after incubation with dabrafenib (50 nM) and trametinib (5 nM). Ectopically expressed MEK1 and MEK2 proteins were tagged with the FLAG and MYC epitopes, respectively. ( b ) Transduced SKMel28 cells were seeded at low density and 24 h after seeding were treated with the indicated concentrations of dabrafenib and trametinib every 72–96 h. Colonies were stained with crystal violet 10 days post transduction. Photographs are representative of at least two independent transduction experiments. Full size image Exome analysis and mutations affecting MAPK, PI3K and other pathways We also sequenced the exomes of eight matched pre-treatment and Prog melanoma pairs, including patient C4 who had unknown mechanisms of resistance and MAPK reactivation ( Table 1 ; Fig. 1 ). All tumours retained the BRAF V600 mutation, and mutant BRAF allele frequency gains from pre-treatment to Prog tumour were significant in four patients (C1, C4, C7 and C10), two of which (patients C7 and C10) showed substantial BRAF gene amplification (mutant and wild type) by quantitative PCR (qPCR) and the other two showing diploid levels of the BRAF gene by qPCR. The exome-sequencing data were consistent with our RT–PCR Sanger sequencing resistance data, except for patient C1 who displayed heterogeneity of the MEK1 G128D mutation; this mutation was not present in the portion of the Prog tumour that was exome sequenced. The MEK2 E207K mutation identified in the Prog from patient C5 was evident in the next generation sequence data ( Supplementary Fig. 2 ), but was not called due to low-quality value ( Supplementary Fig. 2 ). To identify alterations that may diminish response to MAPK inhibition, we cross-referenced recurrently mutated genes in the COSMIC database, genes in the PI3K (KEGG ID:hsa04151) and MAPK (KEGG ID:hsa04010) pathways and genes purported to modulate MAPK inhibitor response [8] , [9] , [19] , [20] , [21] , [22] ( Fig. 1 ; Supplementary Table 1 ). Novel Prog-specific mutations were uncommon, although gains in mutant allele frequency from pre-treatment to Prog were seen in most patients ( Fig. 1 ; Supplementary Table 1 ). Five patients (patients C2, C3, C5, C6 and C10) had tumours with alterations within the PI3K-AKT-mTOR pathway. The activating AKT3 E17K mutation [23] was identified in matched pre-treatment and Prog biopsies derived from patient C5 and the PTEN I33del (ref. 24 ) and PTEN K164fs (COSMIC) alterations were found in melanomas derived from patients C3 and C6, respectively. Uncharacterized mutations affecting AXL (E818K), PTEN (P169S) and SOS1 (R826*) were identified in matched pre-treatment and Prog biopsies derived from patients C3, C6 and C10, respectively. Oncogenic mutations activating the GTPase RAC1 (P29S and P29L) [25] , [26] , [27] were found in matched pre-treatment and Prog melanomas derived from patients C5 and C6. Six patients (patients C1, C3, C4, C5, C6 and C10) had tumours with alterations potentially affecting key proteins of the cell cycle. Melanoma-associated inactivating mutations affecting p16 INK4a (c150+1G>A splice variant, P114L and P81L (refs 28 , 29 ), patients C5, C6 and C10) and previously unidentified missense RB1 variants (I227N, patient C3; S463L, patient C6; and R656W, patient C5) were also found in the pre-treatment and Prog tumours. Alterations potentially affecting the p53 pathway, including a novel MDM2 missense variant (Q414H, patient C4) and the inactivating p53 V218G mutation (patient C1) [30] , were also found in pre-treatment and Prog-matching tumours. The glioma-associated neomorphic mutation in the isocitrate dehydrogenase 1 gene (IDH1 R132C ; refs 31 , 32 ) was identified in the baseline and progressing melanomas derived from patient C10. Patient C7 had no PI3K-AKT alterations identified by exome sequencing in pre-treatment and Prog tumours, yet displayed early resistance with BRAF amplification as the Prog-specific mechanism of resistance. Other alterations identified in both pre-treatment and Prog tumours included novel variants affecting MET, EGFR, SOS2 and RAC2 ( Supplementary Table 1 ). We also confirmed that PI3K-AKT signalling, as evidenced by AKT phosphorylation, correlated with AKT3 E17K /RAC1 P29S mutations and RAC1 P29L /PTEN K164fs mutations in matching tumours derived from patients C5 and C6, respectively ( Fig. 3 ), indicating that AKT activation was present before, during and on combiDT therapy progression. In contrast, AKT phosphorylation was low in the tumours derived from patient C1, who had no detectable alterations activating the PI3K-AKT pathway. Thus, despite the potential importance of this parallel signalling pathway for escape from MAPK inhibition, we did not identify any Prog-specific exome alterations affecting the PI3K-AKT-mTOR network in these CombiDT-resistant tumours. This study describes the largest set of metastatic melanoma patients analysed for resistance mechanisms to combined treatment with BRAF and MEK inhibitors. Most of these patients responded poorly to CombiDT (median tumour reduction was 35%, RECIST response rate 50%) and progressed early (median PFS 3.6 months) when compared with those previously reported [1] . These patients represent a subgroup with early resistance and are in particular urgent need of new, more effective treatment strategies. Nearly all Prog tumours (9/11, 82%) had an identified mechanism of resistance that reactivated MAPK signalling and was not detected in the matched pre-treatment biopsy. This compares with our previous report on resistance to BRAF inhibitor monotherapy in which only 50% of BRAF inhibitor Prog tumours had an identified resistance mechanism and early resistance was associated with continued MAPK inhibition, rather than reactivation [7] . Reactivation of the MAPK pathway occurred primarily via alterations affecting the drug targets (that is, BRAF copy number gains and MEK2 mutations). Although BRAF gene amplification and MEK mutations were also identified in melanomas resistant to BRAF inhibitor monotherapy [7] , [8] , [9] , [10] , [13] , our data show that the upregulation of MAPK signalling was substantially greater in melanomas resistant to CombiDT compared with melanomas resistant to BRAF inhibitor monotherapy. This was most evident when comparing ratios of Prog/pre-treatment BRAF copy number. BRAF amplifications and MAPK output were significantly elevated in the CombiDT-resistant tumours. The significant role of MAPK signalling output in conferring resistance was also evident when analysing BRAF-splice isoforms. The level of MAPK signalling driven by these truncated BRAF proteins was lower relative to that seen with BRAF amplifications, and insufficient to confer trametinib resistance. The recent identification of a BRAF-splice isoform lacking exons 2–10 in a single CombiDT-resistant melanoma suggests that additional genetic alterations may have contributed to drug resistance in that sample [16] . Despite the very high level of mutations in melanomas [19] , [22] , [33] , it is salutary that these tumours retain such high dependency on MAPK activity. The predominance of MAPK reactivation in tumours progressing on CombiDT is unexpected and carries important implications for future clinical trial design strategies in these patients. The abundance of BRAF amplifications is of particular note as ERK inhibitors are active in the context of BRAF copy number gains [34] , including in models resistant to combined BRAF and MEK inhibition [14] . Furthermore, these data suggest that, in unselected patients with CombiDT failure, drug combinations involving PI3K/AKT inhibition (for example, NCT 01902173; ref. 35 ) may prove less successful than additional therapies inhibiting MAPK at multiple nodes, such as those targeting MEK, ERK and possibly CDK4 (NCT01777776, NCT01543698). Although trametinib shows similar inhibitory activity towards the MEK1 and MEK2 proteins in in vitro ERK kinase assays [36] , we observed a preponderance of MEK2 mutations rather than MEK1 mutations in CombiDT-resistant Progs. The fact that the MEK2 C125S mutation and not the homologous MEK1 C121S conferred robust resistance to combination therapy in our preclinical models highlights the functional differences between these highly homologous kinases. Previous reports indicating that MEK2, rather than MEK1, can escape inhibition by the allosteric MEK inhibitor AZD6244 (ref. 37 ) and that MEK2 is the more potent ERK activator [38] , [39] are consistent with our data and recent reports of MEK2 mutations in CombiDT-resistant melanomas [16] , [17] . Current data suggest that ERK activity is gradually restored in the presence of BRAF and MEK inhibitors via receptor tyrosine kinase reprogramming driven by the loss of suppressive feedback regulation [11] , [37] , [40] . The reactivation of ERK promotes the phosphorylation of MEK1 at the negative regulatory Thr292 residue and this facilitates MEK1 inactivation via the dephosphorylation of the activating serine residues [41] , [42] . In contrast, MEK2, which lacks the threonine-negative regulatory site, remains phosphorylated at the activation loop serines in the presence of ERK activity. Activated, phosphorylated MEK proteins also have a significantly lower affinity for trametinib [37] . We are currently exploring the impact of these phosphorylation events on the activity of the MEK1 C121S and MEK2 C125S proteins. Despite the potential importance of the PI3K-PTEN-AKT signalling pathway for escape from MAPK inhibition, we did not identify Prog-specific genetic alterations affecting this pathway. Instead, many tumours carried pre-existing genetic variants, including RAC1, PTEN and AKT3 mutations that activate the PI3K-PTEN-AKT cascade. Consequently, although the sole activation of PI3K activity may not be sufficient to confer CombiDT resistance, we predict that PI3K activity modulates tumour responses to MAPK inhibitors and contributes to early resistance, and that combination MAPK and PI3K/AKT inhibition may be best administered upfront to delay the emergence of resistance [35] . Preclinical data have confirmed that PI3K activation (via NRAS mutations and receptor tyrosine kinase activation) diminished melanoma cell responses to combination BRAF and MEK inhibitors [14] . The hotspot RAC P29S mutation also confers resistance to RAF and MEK inhibitors [26] . Mutations affecting p16 INK4a were also found at baseline and inactivation of this tumour suppressor was associated with a shorter PFS in patients treated with dabrafenib [43] . Loss of p16 INK4a , PTEN and pRb also contributed to intrinsic BRAF inhibitor and MEK inhibitor resistance in vitro [44] , [45] . This cohort was distinguished by the presence of BRAF V600K -mutant melanoma in 50% of patients, a mutation that is present in 6–30% of melanoma tumours [46] , [47] . Patients with BRAF V600K and the more common BRAF V600E -mutant melanoma show significant responses to BRAF inhibitor and combination therapy [1] , [48] , and, although some studies suggest that dabrafenib may be less active in BRAF V600K -mutant melanoma compared with BRAF V600E -mutant disease [48] , [49] , [50] , the response rate, median PFS and OS in vemurafenib-treated patients were similar between the two BRAF genotypes [51] . This study suggests that the genetic effectors mediating acquired resistance to combination BRAF and MEK inhibitors may not be as diverse as those seen with BRAF inhibitor monotherapy. Perhaps, this is not surprising as the simultaneous inhibition of BRAF and MEK1/2 may negate many MAPK resistance effectors signalling above MEK. Surprisingly, MAPK-independent mechanisms of resistance were not acquired at a higher frequency than that in single BRAF inhibitor resistance, suggesting that patients progressing on combination dabrafenib/trametinib therapy may be responsive to drug combinations targeting multiple members of the MAPK pathway and its downstream targets including ERK and CDK4. Durable responses in BRAF-mutant melanoma patients may require combination first-line therapy that selectively inhibits multiple proliferative and survival pathways. Patients, treatment and assessments Patients included in this study had BRAF V600 -mutant metastatic melanoma, had not received prior immunotherapy and were treated with dabrafenib plus trametinib (CombiDT) as part of phase I/II or III clinical trials [1] (NCT01584648, NCT01597908). The majority of patients received maximal recommended daily doses of dabrafenib (300 mg) plus trametinib (2 mg; Table 1 ). Nine of 10 patients had a pre-treatment biopsy and all patients had at least one progressing melanoma metastasis (Prog) resected. Initial Prog lesions were resected within 6 weeks of RECIST-determined disease progression. Subsequent additional Prog biopsies were procured from patients remaining on CombiDT treatment beyond progression. Clinical outcome was assessed using PFS and OS from commencement of CombiDT and RECIST-defined response [52] . Informed consent was obtained for each patient under approved Human Research Ethics Committee protocols. Melanoma tissue samples Fresh melanoma samples were macrodissected by a pathologist and enriched tumour portions snap frozen. Frozen tumour sections were cut, stained with hematoxylin and eosin and scored for the following parameters: % non-tumour cells, % necrosis, degree of pigmentation, predominant cell shape and cell size of the most cellular portion of tumour [53] . Tumour foci were carefully macrodissected utilizing the marked frozen section as a guide to meet minimum criteria for tumour cell content (>80%) and amount of necrosis (<30%). High-percentage tumour content was verified by examining post-macrodissection frozen section slides. Total RNA was extracted from 10 to 20 mg of tumour. Tissue samples were homogenized using a high-speed agitation Polytron blender (Kinematica, Luzern, Switzerland) in the presence of Trizol (Life Technologies, Carlsbad, CA, USA). Following homogenization, chloroform was added and the sample centrifuged. The upper phase was removed and mixed with 70% ethanol. The RNA was then isolated and purified with an RNeasy purification kit with DNase I digestion on the column (Qiagen, Valencia, CA, USA). The quality of the RNA preparations was assessed using a Agilent 2100 Bioanalyser (Agilent Technologies, Palo Alto, CA, USA). The extracted total RNA was of high quality (RNA integrity number: 8–10). Analysis of resistance mechanisms and gene expression analysis The expression of BRAF-splice variants, the complete coding sequence of MEK1 , MEK2 and NRAS complementary DNAs and the 5′ half of the AKT1 cDNA were examined using an RT–PCR screen [7] . Reverse transcription reactions were performed using the Superscript III First-Strand Synthesis kit (Invitrogen) with the oligo dT primer. The MEK1 , MEK2 , NRAS and AKT1 gene products were each amplified from cDNA using Taq polymerase (Fisher Biotech, Wembley, WA, Australia) and BRAF cDNA was amplified with Pfx polymerase (Life Technologies). Amplification and sequencing primers are listed in Supplementary Table 2 . PCR products were purified using QIAquick PCR purification kit (Qiagen, Limburg, Netherlands) followed by Sanger sequencing on the 3730xl DNA Analyser (AGRF, Westmead, NSW, Australia). BRAF relative copy number was determined by qPCR using the Corbett Rotor-Gene 6000 (ref. 54 ). Gene expression analysis was performed on matched pre-treatment ( n =9) and Prog ( n =10) biopsies derived from nine patients, using the Sentrix HumanHT12 v.4.0 Expression BeadChip (Illumina, San Diego, CA, USA). Complementary RNA amplification and labelling with biotin were performed using the Illumina TotalPrep RNA amplification kit (Ambion, Austin, TX, USA) according to the manufacturer’s instructions starting with 250 ng total RNA [7] . Three responding (that is, shrinking) melanoma samples taken early during BRAF inhibitor monotherapy ( n =2) or combination BRAF and MEK inhibitor therapy ( n =1; EDT; 2–7 days after therapy initiation) were also included in these gene expression analyses. Reproducibility of gene expression data was confirmed by including technical replicates, in which RNA was independently amplified and hybridized on different arrays and on separate days. Clustering using GenomeStudio (Illumina) confirmed that each replicate showed <1.2% variation. The microarray platform and data have been submitted to the Gene Expression Omnibus public database at the National Center for Biotechnology Information, following the minimum information about microarray gene experiment guidelines. The accession code is GSE61992. Exome sequencing Exome sequencing was performed on patient-matched Pre and Prog melanoma tissues. Exonic DNA was enriched using the Illumina TrueSeq technology, targeting 62 Mb encompassing protein-coding regions ( Supplementary Table 3 ), and sequenced on an Illumina HiSeq2000. We aligned the read pairs to the reference human genome (hg19) using Burrows-Wheeler Aligner (BWA) [55] , removed duplicates with Picard and applied GATK indel realignment and base quality recalibration [56] . Single-nucleotide variants and small insertion/deletions (INDELS) were detected by SAMTools [57] . To generate a list of high-quality variants, we removed low-coverage variants (single-nucleotide polymorphism quality <30, read <30) and eliminated variants annotated as common polymorphisms or in the 1000 Genomes Project. We used Ingenuity Variant Analysis ( http://www.ingenuity.com ) to compare the remaining mutations between the pre-treatment and Prog samples from each patient to detect oncogenic variants and Prog-specific cancer-driver mutations. When a somatic mutation was present in both the pre-treatment and Prog samples for a given patient, Fisher’s exact test was used to determine whether the difference in allele frequency was statistically significant. Cell culture and constructs Short-term cultures were established from a subset of patients by mechanically processing tissue in Dulbecco’s Modified Eagle Medium (DMEM)/10% fetal calf serum (FCS) containing 100 U ml −1 penicillin and 100 μg ml −1 streptomycin (Gibco BRL). The clarified cell suspension was maintained in DMEM/10% FCS containing penicillin and streptomycin (Gibco). Contaminating fibroblasts were removed by treating cultures with 100 μg ml −1 G418 (Gibco) as required [58] . Cells were grown in DMEM with 10% FCS and glutamine (Gibco BRL) and cultured in a 37 °C incubator with 5% CO 2 . Stocks of dabrafenib (supplied by Active Biochem, Maplewood, NJ, USA) and trametinib (Selleck Chemicals, Houston, TX, USA) were made in dimethyl sulfoxide. Cell authentication was confirmed using the StemElite ID system from Promega. Lentiviruses were produced in HEK293T cells using expression vectors encased in viral capsid encoded by three packaging plasmids as described earlier [59] , [60] . Cells were infected using a multiplicity of infection of 1–5 to provide an efficiency of infection above 90%. Wild-type and mutant FLAG-tagged MEK1 and MYC-tagged MEK2 constructs were each cloned into the pCDH-CuO-MCS-EF1-CymR-PURO and plenti6.3/T0/V5-DEST lentiviral vectors, respectively. Clonogenic and pharmacological growth assays Approximately 96 h post-transduction, melanoma cells were seeded at 25,000 cells per well onto six-well culture plates and allowed to grow for 24 h followed by the desired treatment. Cells were then washed twice with ice-cold PBS and fixed with ice-cold methanol for 1 min. After aspirating methanol from plates, 0.1% crystal violet (Sciencelab.com, TX, USA) solution was added and the plate was incubated at room temperature for 5 min. Distilled water was used to rinse the plate. Pharmacological growth inhibition assays were performed using 1–2 × 10 3 cells per well in 96-well plates and 24 h after seeding, serial dilutions of each inhibitor were added to cells. Cells were incubated for an additional 72 h and cell viability was measured using the Cell proliferation Aqueous MTS assay (Promega) on a VICTOR [2] Multilabel counter (PerkinElmer) [58] . Western blotting and immunohistochemistry Total cellular proteins were extracted at 4 °C using radioimmunoprecipitation assay lysis buffer containing protease inhibitors and phosphatase inhibitors (Roche). Proteins (40 μg) were resolved on 12% SDS–polyacrylamide gels and transferred to Immobilon-P membranes (Millipore). Western blots were probed with the following antibodies: total ERK (1:2000; 137F5; Cell Signaling, Danvers, MA, USA), phosphorylated ERK (1:2000; E-4; Santa Cruz, Santa Cruz, CA, USA), MYC (1:1000; A-14; Santa Cruz), FLAG (1:1000; Sigma-Aldrich, St Louis, MO, USA), MEK1/2 (1:2000; L38C12, Cell Signaling), phosphorylated pRb (1:500; Cell Signaling) and β-actin (1:6000; AC-74; Sigma-Aldrich). Immunohistochemical staining of selected matched formalin-fixed, paraffin-embedded melanoma specimens using phosphorylated AKT (1:75; CS-3787; Cell Signaling) was performed on a Dako Autostainer Plus (Dako, Glostrup, Denmark), utilizing the EnVision FLEX, High pH visualization system (K8024, Dako) according to the manufacturer’s protocol. Sections (4 μm) were baked at 58 °C for 60 min, then underwent deparaffinization and antigen retrieval using the heat-induced epitope retrieval method with Envision Flex Target Retrieval Solution (High pH) in a PT link unit (Dako). Antibody detection was performed using the Dako Envision Flex HRP (Dako) and visualized using 3,3′-diaminobenzidine (Dako), and the slides were counterstained with Harris’s hematoxylin [7] . Statistical analysis The Kaplan–Meier method was used to calculate median OS and PFS from the date of commencement on combination therapy, together with the Cox–Mantel log-rank test to calculate statistical significance where appropriate. Confidence intervals for proportions were calculated without continuity correction. The Mann–Whitney U -test was used to compare medians for nonparametric groups. How to cite this article: Long, G. V. et al . Increased MAPK reactivation in early resistance to dabrafenib/trametinib combination therapy of BRAF-mutant metastatic melanoma. Nat. Commun. 5:5694 doi: 10.1038/ncomms6694 (2014). Accession codes : Exome sequence data derived from pre-treatment and Prog melanoma tumours have been deposited in the European Nucleotide Archive core database under the accession code PRJEB7503 . The microarray data have been deposited in the Gene Expression Omnibus public database at the National Center for Biotechnology Information, under the accession code GSE61992 .